Export of a single drug molecule in two transport cycles by a multidrug efflux pump Secondary multidrug transporters use ion concentration gradients to energize the removal from cells of various antibiotics. The Escherichia coli multidrug transporter MdfA exchanges a single proton with a single monovalent cationic drug molecule. This stoichiometry renders the efflux of divalent cationic drugs energetically unfavourable, as it requires exchange with at least two protons. Here we show that surprisingly, MdfA catalyses efflux of divalent cations, provided that they have a unique architecture: the two charged moieties must be separated by a long linker. These drugs are exchanged for two protons despite the apparent inability of MdfA to exchange two protons for a single drug molecule. Our results suggest that these drugs are transported in two consecutive transport cycles, where each cationic moiety is transported as if it were a separate substrate. We propose that secondary transport can adopt a processive-like mode of action, thus expanding the substrate spectrum of multidrug transporters. Multidrug resistance (Mdr) transporters are ubiquitous membrane proteins that provide cells with defense against various cytotoxic compounds. They function as multispecific efflux pumps, each able to expel a broad spectrum of chemically dissimilar drugs out of the cell [1] . Bacteria typically harbour numerous Mdr transporter-encoding genes in their genomes, which function as secondary transporters driven by the proton motive force [2] . Bacterial Mdr transporters exist in several phylogenetically and mechanistically distinct protein families [3] . Of those, H + /multidrug antiporters of the Major Facilitator Superfamily (MFS) comprise the largest group [1] . Different MFS Mdr transporters work with distinct proton antiport stoichiometries. Although a stoichiometry of one proton per drug was observed with MdfA from E. coli [4] , [5] , QacA from Staphylococcus aureus and LmrP from Lactococcus lactis use stoichiometries of up to 2 and 3, respectively [6] , [7] . Recent progress has shed light on the mechanism of proton transport by MdfA, in which a membrane-embedded acidic residue facilitates proton binding and transport [4] . Mutagenesis experiments indicate that increasing the proton stoichiometry of MdfA from 1 to 2 is possible by introducing an additional acidic residue in a number of membrane-embedded locations [8] . LmrP, which works with a stoichiometry of up to three protons, contains three membrane-embedded acidic residues; each functions as a module that facilitates the transport of a single proton [7] . As shown recently, the stoichiometry of one proton per drug renders MdfA inactive in efflux of divalent cationic (dicationic) drugs, which require import of two protons per transport cycle [8] . The underlying reason is that such an antiport reaction (export of drug 2+ in exchange for a single H + ) involves net charge efflux that opposes the membrane potential (Δ ψ , interior negative). Indeed, MdfA mutants that are capable of pumping out two protons per drug are able to confer resistance against dicationic drugs [8] . Surprisingly, we show here that also wild-type MdfA can actively pump certain dicationic drugs. However, in this case the dicationic drugs must have a distinct chemical architecture, in which the two cationic moeities are separated by a long linker. Our studies suggest that each of these drugs is transported in two successive transport cycles, where the cationic moieties are treated as if they were separate monocationic substrates. This unexpected mechanism expands the Mdr spectrum of MdfA towards a new group of dicationic drugs and indicates that secondary transporters can operate in a processive-like manner. MdfA confers resistance against unique dicationic drugs During our characterization of the drug recognition spectrum of MdfA, we were surprised to find that it confers resistance against the toxic dicationic compound dequalinium (Dq). The chemical structure of Dq reveals that it contains two identical cationic pharmacophores separated by a long, ten-carbon chain linker ( Fig. 1a ). To examine whether these characteristics of Dq (symmetry and spacer length) are relevant to the unexpected activity, we challenged MdfA with several dicationic drugs ( Fig. 1a ). In some of these compounds, both positive charges are relatively close (4′,6-diamidino-2-phenylindole (DAPI), diminazene (Dmn) and methyl viologen), while in others the positive charges are separated by long linkers (Dq, chlorhexidine (Chx) and pentamidine (Pent)). For simplicity, we term the two groups of compounds SDCs ( s hort d icationic c ompounds) and LDCs ( l ong d icationic c ompounds), respectively. Strikingly, when challenged against all these drugs, we observed that MdfA could only protect E. coli against LDCs, demonstrating that symmetry alone is not sufficient and that the linker length is important ( Fig. 1b ). 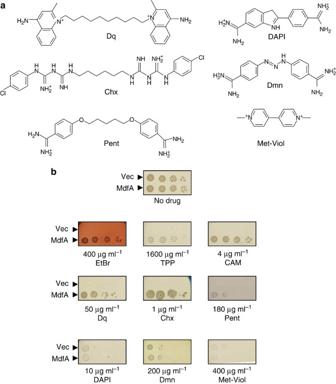Figure 1: MdfA confers resistance only against a unique class of symmetric dicationic compounds (LDC). (a) Structures of the tested dicationic drugs. Left: long dicationic compounds (LDCs): dequalinium (Dq), chlorhexidine (Chx) and pentamidine (Pent). Right: short dicationic compounds (SDCs): 4′,6-diamidino-2-phenylindole (DAPI), diminazene (Dmn) and methyl viologen (Met-Viol). (b) Growth ofE. coliUTmdfA::kanexpressing MdfA from a multicopy plasmid (or harboring empty vector) on solid media supplemented with the indicated drugs. Tenfold serial dilutions of cells were plated from left to right and grown overnight. The upper panels show controls of growth in the absence of drug or in the presence of previously known monocationic (TPP/ethidium bromide (EtBr)) or neutral (CAM) MdfA substrates. The experiments were repeated at least three times and the results shown are representative. Figure 1: MdfA confers resistance only against a unique class of symmetric dicationic compounds (LDC). ( a ) Structures of the tested dicationic drugs. Left: long dicationic compounds (LDCs): dequalinium (Dq), chlorhexidine (Chx) and pentamidine (Pent). Right: short dicationic compounds (SDCs): 4′,6-diamidino-2-phenylindole (DAPI), diminazene (Dmn) and methyl viologen (Met-Viol). ( b ) Growth of E. coli UT mdfA::kan expressing MdfA from a multicopy plasmid (or harboring empty vector) on solid media supplemented with the indicated drugs. Tenfold serial dilutions of cells were plated from left to right and grown overnight. The upper panels show controls of growth in the absence of drug or in the presence of previously known monocationic (TPP/ethidium bromide (EtBr)) or neutral (CAM) MdfA substrates. The experiments were repeated at least three times and the results shown are representative. Full size image The resistance conferred by MdfA suggests that unlike SDCs, LDCs are actively extruded by the transporter. To test this, we characterized the ability of MdfA to prevent Dq accumulation in vivo in whole cells. The fluorescence of Dq is quenched when it enters cells ( Fig. 2a ) and can be de-quenched on lysis of cells that accumulated Dq ( Fig. 2b ). 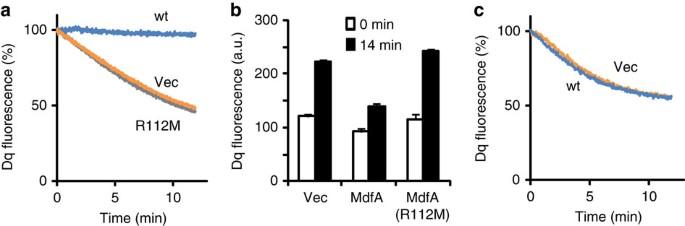Figure 2: MdfA-mediated Dq transport. (a) Characterization of Dq accumulation byE. coliUTL2mdfA::kanoverexpressing MdfA or its inactive mutant MdfA(R112M), or cells harbouring an empty plasmid. (b) Quantitative Dq accumulation. Cells were suspended in buffer containing glucose and Dq (1 μM), and allowed to accumulate Dq for 0 or 14 min. Dq fluorescence in these cells was determined after the cells were harvested and lysed, relieving their fluorescence quenching effect. Error bars indicate range of duplicate measurements. (c) Dq accumulation by control or MdfA-expressing cells in the presence of 0.8 mM CAM. (a,c) The experiments were repeated at least three times and the results shown are representative. Figure 2a,b show that expression of MdfA from a multicopy plasmid indeed prevented intracellular accumulation of Dq compared with cells harbouring an empty vector or expressing the inactive mutant MdfA(R112M) [4] , [9] . In addition, extrusion of Dq was completely inhibited when another substrate of MdfA, chloramphenicol (CAM), was added as a competitor ( Fig. 2c ), as shown previously for another MdfA substrate [10] . These results suggest that MdfA mediates active transport of Dq. Figure 2: MdfA-mediated Dq transport. ( a ) Characterization of Dq accumulation by E. coli UTL2 mdfA::kan overexpressing MdfA or its inactive mutant MdfA(R112M), or cells harbouring an empty plasmid. ( b ) Quantitative Dq accumulation. Cells were suspended in buffer containing glucose and Dq (1 μM), and allowed to accumulate Dq for 0 or 14 min. Dq fluorescence in these cells was determined after the cells were harvested and lysed, relieving their fluorescence quenching effect. Error bars indicate range of duplicate measurements. ( c ) Dq accumulation by control or MdfA-expressing cells in the presence of 0.8 mM CAM. ( a , c ) The experiments were repeated at least three times and the results shown are representative. Full size image MdfA binds both LDCs and SDCs How does MdfA distinguish between the two groups of dicationic drugs? One possibility is that MdfA cannot bind SDCs. To test this, we measured the ability of SDCs and LDCs to compete with a radiolabelled substrate, the monovalent [ 3 H]-tetraphenylphosphonium (TPP), for binding to MdfA. The results show that with the exception of methyl viologen, all the tested dicationic compounds are able to outcompete [ 3 H]-TPP-binding in a concentration-dependent manner ( Fig. 3 ). The concentration dependency suggests that MdfA has similar affinities to these compounds as those reported for other known substrates [10] . Thus, the reason for the discrimination between the two types of dicationic substrates does not stem from differences in their ability to bind the transporter. 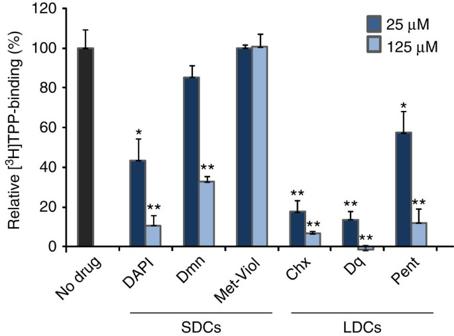Figure 3: MdfA binds both groups of dicationic drugs (LDCs and SDCs). [3H]-TPP binding by wild-type MdfA and its inhibition by addition of increasing concentrations (25 or 125 μM) of dicationic drugs. Error bars indicate s.d. of triplicate measurements (*P<10−2; **P≤10−4compared with the no drug sample, one tailedt-test). The experiments were repeated at least three times and the results shown are representative. Figure 3: MdfA binds both groups of dicationic drugs (LDCs and SDCs). [ 3 H]-TPP binding by wild-type MdfA and its inhibition by addition of increasing concentrations (25 or 125 μM) of dicationic drugs. Error bars indicate s.d. of triplicate measurements (* P <10 −2 ; ** P ≤10 −4 compared with the no drug sample, one tailed t -test). The experiments were repeated at least three times and the results shown are representative. Full size image MdfA catalyses LDC/proton antiport To further evaluate the indication that MdfA actively exports LDCs, we performed transport experiments with everted membrane vesicles. As MdfA-catalysed active efflux relies on drug/proton antiport, we measured substrate-dependent proton transport by MdfA in vesicles from cells expressing MdfA or harbouring an empty vector. The proton concentration gradient (ΔpH) across these membranes was followed by measuring the fluorescence of a ΔpH-sensitive indicator, 9-amino-6-chloro-2-methoxyacridine (ACMA). Energization of everted membrane vesicles by D , L -lactate oxidation generated a ΔpH (acidic inside) as observed by quenching of ACMA fluorescence ( Fig. 4 ). The generated ΔpH was fully dissipated by adding the proton conducting uncoupler carbonyl cyanide m -chlorophenyl hydrazone ( Fig. 4 ). Addition of substrates from the LDCs group (Dq, Pent or Chx) or the control monocationic substrate TPP partially dissipated ΔpH only in membranes expressing MdfA ( Fig. 4 , compare left and right panels). Thus, MdfA indeed catalyses proton/LDC exchange. In contrast, addition of the SDC compound Dmn did not trigger proton translocation. Notably, this assay is not quantitative because calculating the amount of protons transported by MdfA in the presence of different compounds might be complicated by other factors such as the ability of the different substrates to distribute across the membrane via MdfA-independent routes. Consequently, as expected, the magnitude to which different substrates affect ΔpH (as reflected by the fluorescence change) did not show any correlation with the charges on the substrates. 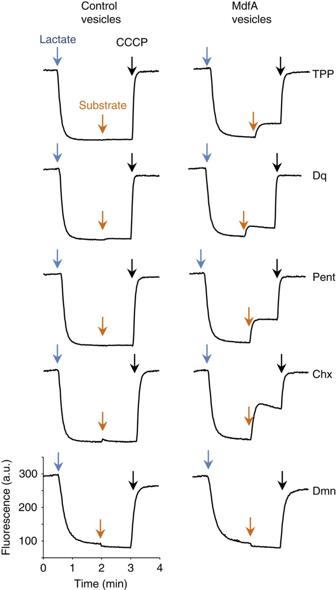Figure 4: Proton transport by control or MdfA-containing everted membrane vesicles. The transmembrane ΔpH was followed by measuring ACMA fluorescence. Lactate (added after 0.5 min, blue arrow) and carbonyl cyanidem-chlorophenyl hydrazone (CCCP; after 3 min, black arrow) were used to generate or abolish ΔpH, respectively. Substrates were added at 2 min (orange arrow), in the following concentrations: TPP (125 μM), Dq (25 μM), Pent (125 μM), Chx (25 μM) and Dmn (12.5 μM). The experiments were repeated at least three times and the results shown are representative. Figure 4: Proton transport by control or MdfA-containing everted membrane vesicles. The transmembrane ΔpH was followed by measuring ACMA fluorescence. Lactate (added after 0.5 min, blue arrow) and carbonyl cyanide m -chlorophenyl hydrazone (CCCP; after 3 min, black arrow) were used to generate or abolish ΔpH, respectively. Substrates were added at 2 min (orange arrow), in the following concentrations: TPP (125 μM), Dq (25 μM), Pent (125 μM), Chx (25 μM) and Dmn (12.5 μM). The experiments were repeated at least three times and the results shown are representative. Full size image MdfA-catalysed transport of LDCs is electroneutral As explained earlier, it is energetically unfavourable for any antiporter to export dicationic substrates by using a proton/substrate stoichiometry of 1, as the resulting reaction would involve net export of a positive charge against the membrane potential. Therefore, as wild-type MdfA usually works with a stoichiometry of 1, the transport of LDCs is enigmatic. To better understand this important phenomenon, we characterized the electrogenicity of the LDCs transport reactions. We assumed that MdfA may use a proton/dicationic substrate stoichiometry of ⩾ 2, resulting in electroneutral or electrogenic transport, respectively, which involves no export of a net positive charge(s). As a first attempt to probe transport energetics in living cells, we determined the effect of the external pH on MdfA-mediated resistance to neutral, monocationic and LDC drugs. When the external pH rises above the intracellular level of ~7.6, the pH gradient across the membrane (ΔpH) reverses its direction and becomes acidic inside relative to outside [11] . Thus, electroneutral transport reactions, which rely energetically only on ΔpH, become unfavourable. In contrast, electrogenic transport reactions are still supported by the electrical potential (Δψ, interior negative) [5] . Our results confirmed previous experiments with MdfA [5] , which showed that resistance against the neutral substrate CAM is driven by both components of the electrochemical potential (Δψ and ΔpH), whereas resistance against the monovalent cation ethidium bromide is solely dependent on the ΔpH ( Fig. 5a ). 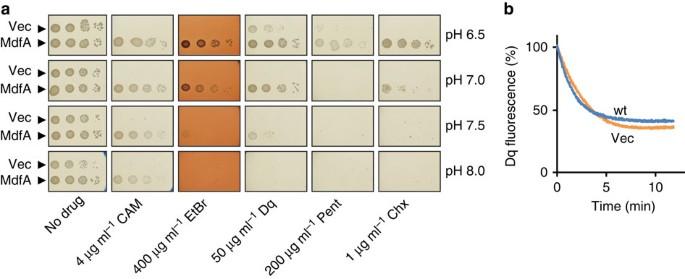Figure 5: pH dependence of MdfA-mediated Mdr. (a) pH-dependent drug resistance assay. The experiment was done as inFig. 1b, with a pH-buffering agent (Bis-Tris-Propane) added to the medium to generate the pH indicated to the right. (b) Accumulation of Dq in ΔpH-dissipated cells. Dissipation of ΔpH was achieved by conducting the assay at pH 8 in the presence of 2 μM nigericin. The membranes were permeabilized to nigericin by an EDTA-ethanol treatment, which did not affect the assay when the ΔpH was not dissipated. The experiments were repeated at least three times and the results shown are representative. Figure 5a also shows clearly that MdfA-mediated resistance against LDCs (Dq, Chx and Pent), just like ethidium bromide, is pH dependent, suggesting that the transport reaction with these drugs is electroneutral. To further assess the proposed electroneutral mode of antiport in the case of LDCs, we measured Dq accumulation in living cells depleted of the ΔpH (by addition of the ionophore nigericin and external pH 8). These conditions make drug efflux possible only if it can be driven by Δψ. However, Fig. 5b shows that this was not the case and MdfA could not catalyse antiport of Dq when Δψ (interior negative) is the sole driving force. Figure 5: pH dependence of MdfA-mediated Mdr. ( a ) pH-dependent drug resistance assay. The experiment was done as in Fig. 1b , with a pH-buffering agent (Bis-Tris-Propane) added to the medium to generate the pH indicated to the right. ( b ) Accumulation of Dq in ΔpH-dissipated cells. Dissipation of ΔpH was achieved by conducting the assay at pH 8 in the presence of 2 μM nigericin. The membranes were permeabilized to nigericin by an EDTA-ethanol treatment, which did not affect the assay when the ΔpH was not dissipated. The experiments were repeated at least three times and the results shown are representative. Full size image Taken together, the results indicate that the transport of the dicationic drug Dq is electroneutral and depends solely on the ΔpH. These results are intriguing, because Dq and each of the other LDCs carry two positive charges, meaning that two protons are exchanged for one drug molecule during the antiport. However, as MdfA cannot translocate two protons simultaneously, export of LDCs requires a novel mode of transport (see later). LDC binding triggers release of a single proton from MdfA How does the long linker between the charges in LDCs ( Fig. 1a ) allow transport with an increased proton/drug stoichiometry of 2? Recent studies have indicated that the antiport mechanism of MdfA relies on competition between substrate and proton on binding to the transporter. Monocationic substrates were shown to trigger the release of a single stoichiometric proton from MdfA, in agreement with an antiport stoichiometry of 1 (ref. 4 ). Here, one possible scenario is that the linker in LDCs enables the two cationic moieties to trigger proton release from two distinct proton-binding sites, if those exist in MdfA. We therefore tested whether LDCs compete with only one or maybe two protons for binding. To this end, we compared the amount of protons released from MdfA on binding of the LDCs Dq and Pent with the amount released by binding of the monocationic TPP. Proton release was inferred from an increase in the solution’s acidity, as measured by the fluorescent pH indicator fluorescein [4] . Notably, Chx could not be tested in this assay because it generates high artificial fluorescent signals (not shown). 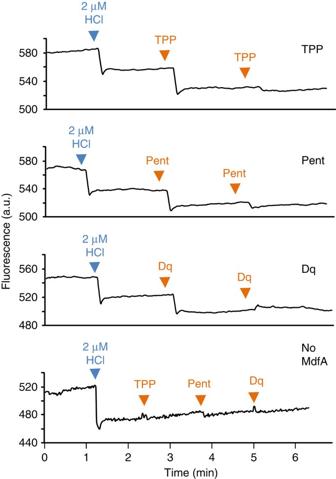Figure 6: Substrate-induced proton release. MdfA was solubilized and purified to homogeneity and dialysed to remove buffering agents. The protein was diluted to 2 μM and the solution acidity was monitored in a time-dependent manner by measuring the pH-sensitive fluorescence of the probe fluorescein. Before the assay, the protein was titrated by NaOH or HCl to a fluorescent signal of ~550 (pH~6.5). Notably, the absence of a buffering agent generates spontaneous slow drifts in the acidity, creating a background signal. The substrate-induced changes are distinguished from the background by their much higher rate of changes. The arrows denote additions of HCl (2 μM), TPP (150 μM), Pent (300 μM) or Dq (50 μM). HCl was added in an MdfA-equimolar amount to reveal the signal expected by a stoichiometric release of a single proton per MdfA molecule. This signal is nearly identical to that of substrates (TPP/Dq/Pent), suggesting that all substrates release a single proton from MdfA. Substrates were added at saturating concentrations. As a control, substrates were added twice to examine the saturability of binding and the related proton release. In addition, substrates did not appreciably affect fluorescence when added to a solution without MdfA (lower panel). The experiments were repeated at least three times and the results shown are representative. Figure 6 shows that despite the differences in transport stoichiometry, the dicationic drugs Dq and Pent, and the monocationic compound TPP, all induced the release of a single stoichiometric proton from MdfA. Thus, it appears that MdfA contains a single proton-binding site. Figure 6: Substrate-induced proton release. MdfA was solubilized and purified to homogeneity and dialysed to remove buffering agents. The protein was diluted to 2 μM and the solution acidity was monitored in a time-dependent manner by measuring the pH-sensitive fluorescence of the probe fluorescein. Before the assay, the protein was titrated by NaOH or HCl to a fluorescent signal of ~550 (pH~6.5). Notably, the absence of a buffering agent generates spontaneous slow drifts in the acidity, creating a background signal. The substrate-induced changes are distinguished from the background by their much higher rate of changes. The arrows denote additions of HCl (2 μM), TPP (150 μM), Pent (300 μM) or Dq (50 μM). HCl was added in an MdfA-equimolar amount to reveal the signal expected by a stoichiometric release of a single proton per MdfA molecule. This signal is nearly identical to that of substrates (TPP/Dq/Pent), suggesting that all substrates release a single proton from MdfA. Substrates were added at saturating concentrations. As a control, substrates were added twice to examine the saturability of binding and the related proton release. In addition, substrates did not appreciably affect fluorescence when added to a solution without MdfA (lower panel). The experiments were repeated at least three times and the results shown are representative. Full size image Dq binds to MdfA with 1:1 stoichiometry Another purely theoretical possibility is that LDCs bind to an MdfA dimer where each MdfA molecule binds one of the separable cationic moieties, thus transporting the substrate cooperatively. We do not favour this possibility because MdfA and other MFS transporters are known to function as monomers [12] , [13] . In addition, the several available structures of MFS members show that the binding sites are located deep within the proteins [14] , [15] , [16] , [17] , [18] and therefore the spacer separating the two cationic moieties of LDCs would not fit the length required for binding to separate transporters in the membrane. Indeed, we saw no evidence for cross-linking of MdfA dimers on Dq binding, when attempting to cross-link with formaldehyde, paraformaldehyde or disuccinimidylsuberate (data not shown). To further examine the binding stoichiometry, we characterized the interaction of purified MdfA protein with Dq. Binding was measured fluorimetrically, by following Dq fluorescence. The results show that on MdfA binding, the fluorescence of Dq is quenched ( Fig. 7a ). This effect is not observed when Dq is mixed with the inactive mutant MdfA(R112M) [4] , or when TPP is added as a competitive inhibitor ( Fig. 7a ). We next determined the affinity of Dq binding to MdfA by two complementary approaches, in which one component (either MdfA or Dq) is kept constant at a low concentration, while the other component is titrated at increasing concentrations. 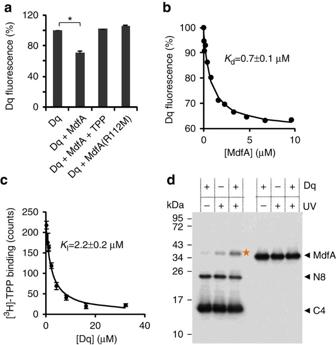Figure 7: Affinity and stoichiometry of Dq binding by purified MdfA. (a) Quenching of 0.2 μM Dq fluorescence by 2 μM wild-type MdfA or MdfA(R112M). Effect of adding 1 mM TPP to the mixture is also shown. Error bars indicate s.d. of triplicate measurements (*P<10−4, two-tailedt-test). (b) Quenching of 0.2 μM Dq fluorescence by increasing MdfA concentrations. The binding of Dq to MdfA was analysed by nonlinear regression fitting (line), yielding the indicatedKd. (c) Inhibition of [3H]-TPP binding to MdfA by increasing Dq concentrations. The results were analysed by non-linear regression fitting (line), yielding the indicatedKI. Error bars indicate s.d. of triplicate measurements. (d) Dq-mediated photoinduced cross-linking of MdfA. Membranes expressing functional split-MdfA (C-terminally tagged N8-His6and C4-His6, left lanes) or wild-type MdfA-His6(right lanes) were incubated in the absence or presence of 100 μM Dq and irradiated with ultraviolet. Proteins were separated by SDS–PAGE and western blotting against the His tag. Cross-linked product of N8 and C4 is indicated by a star. Figure 7b shows the effect of increasing [MdfA] on Dq fluorescence and Fig. 7c shows the competitive inhibition of TPP binding by MdfA, mediated by increasing [Dq]. The two approaches yield comparable dissociation constants, with K d ~0.7 μM for MdfA at ambient temperature measured by Dq fluorescence ( Fig. 7b ) and K I of ~2 μM determined from [ 3 H]-TPP binding-competition experiments at 4 °C ( Fig. 7c ). Notably, both binding curves are hyperbolic, suggesting no cooperativity in binding, consistent with a binding stoichiometry of 1. Figure 7: Affinity and stoichiometry of Dq binding by purified MdfA. ( a ) Quenching of 0.2 μM Dq fluorescence by 2 μM wild-type MdfA or MdfA(R112M). Effect of adding 1 mM TPP to the mixture is also shown. Error bars indicate s.d. of triplicate measurements (* P <10 −4 , two-tailed t -test). ( b ) Quenching of 0.2 μM Dq fluorescence by increasing MdfA concentrations. The binding of Dq to MdfA was analysed by nonlinear regression fitting (line), yielding the indicated K d . ( c ) Inhibition of [ 3 H]-TPP binding to MdfA by increasing Dq concentrations. The results were analysed by non-linear regression fitting (line), yielding the indicated K I . Error bars indicate s.d. of triplicate measurements. ( d ) Dq-mediated photoinduced cross-linking of MdfA. Membranes expressing functional split-MdfA (C-terminally tagged N8-His 6 and C4-His 6 , left lanes) or wild-type MdfA-His 6 (right lanes) were incubated in the absence or presence of 100 μM Dq and irradiated with ultraviolet. Proteins were separated by SDS–PAGE and western blotting against the His tag. Cross-linked product of N8 and C4 is indicated by a star. Full size image To evaluate the results more directly, we conducted Dq-mediated cross-linking of MdfA. Dq is a photoactivatable compound that on ultraviolet irradiation is able to react covalently with nearby residues [19] . The results show that Dq can cross-link a functionally active [20] split mutant of MdfA, in which the 8 amino-terminal (N8) and the 4 carboxy-terminal (C4) transmembrane helices were expressed as separate polypeptides with C-terminal hexahistidine tags ( Fig. 7d ). This indicates that Dq can interact with two separate regions of MdfA, at least transiently. In contrast, Dq could not cross-link two molecules of full-length MdfA ( Fig. 7d ), suggesting that interaction of Dq with an MdfA dimer does not take place. Export of dicationic substrates by other Mdr transporters The results of all the previous experiments support the notion that MdfA translocates two protons in exchange for a single LDC molecule, but probably not simultaneously. This led us to propose another explanation for the increased stoichiometry during transport of LDCs. We hypothesized that MdfA transports these unique drug molecules in two successive transport cycles. According to this scenario, MdfA handles each positively charged group as if it were a separate substrate, which is transported against a proton (see model in Fig. 8 ). 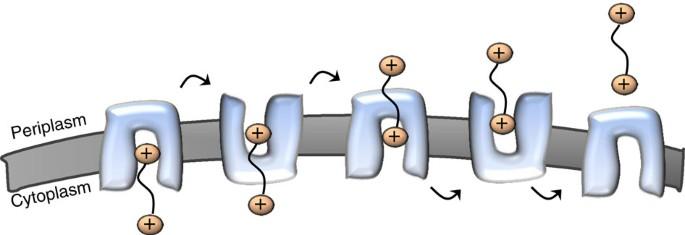Figure 8: Model for transport of divalent cations in two successive transport cycles. The transporter first binds and transports only one cationic moiety (sphere) of the substrate. Once this moiety is expelled, the transporter binds and then transports the second half of the substrate. Each transport cycle is depicted as an interconversion between inward- and outward-facing conformations. Figure 8: Model for transport of divalent cations in two successive transport cycles. The transporter first binds and transports only one cationic moiety (sphere) of the substrate. Once this moiety is expelled, the transporter binds and then transports the second half of the substrate. Each transport cycle is depicted as an interconversion between inward- and outward-facing conformations. Full size image The suggestion that transport of a single substrate proceeds in two consecutive cycles relies only on the substrate properties. Therefore, we reasoned that this ability to transport LDCs might not be unique to MdfA but perhaps shared by other MFS Mdr transporters. To test the generality of this phenomenon, we studied QacA, a different MFS-related Mdr transporter from S. aureus . QacA transports both monocationic and dicationic drugs [21] , and previous studies showed that the activity of QacA against the dicationic drugs depends on an acidic residue at position 323 (ref. 22 ). Neutralizing D323 by mutagenesis interrupted the activity towards dications while retaining active efflux of monocationic drugs [6] . We speculated that a mechanism involving two consecutive transport cycles should enable the D323 mutant of QacA to transport LDCs, but not SDCs. This was tested by drug resistance assays using E. coli harbouring heterologously expressed QacA or QacA(D323C). As expected, the results show that wild-type QacA was able to confer resistance against all tested dicationic drugs (LDCs and SDCs) ( Fig. 9a ). Remarkably, however, although the QacA(D323C) mutant had partially lost its ability to transport SDCs, it retained resistance activity against LDCs (Dq and Chx) ( Fig. 9a ). These results support our hypothesis that a monocationic Mdr transporter can transport dicationic substrates that belong to the LDC group. In support of this notion, previous studies have shown that QacB, a close variant of QacA harbouring a neutral residue at position 323 and consequently lacked activity against most dications, was found to retain activity towards several dicationic drugs. The common denominator of these drugs is that their two cationic moieties are separated by a long linker [6] , [22] , [23] , and meet our criteria for LDCs. 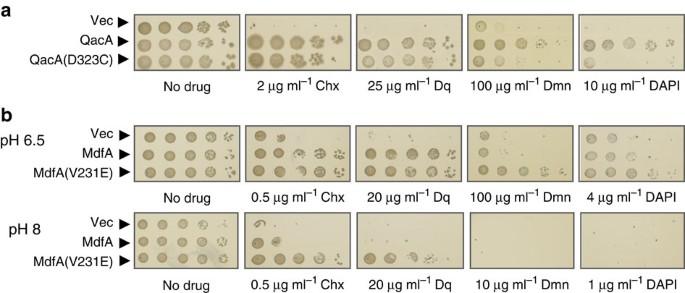Figure 9: Effect of acidic residue substitutions on resistance against dications by QacA and MdfA. The experiments were done as inFigs 1band5. (a) Mdr byE. coliexpressing QacA or its D323C mutant. (b) pH dependence of multidrug resistance byE. coliUTmdfA::kanexpressing MdfA or its V231E mutant. Resistance to Dmn and DAPI at pH 8 was tested at lower drug concentrations than pH 6.5 to make sure that even low-level resistance is not conferred. The experiments were repeated at least three times and the results shown are representative. Figure 9: Effect of acidic residue substitutions on resistance against dications by QacA and MdfA. The experiments were done as in Figs 1b and 5 . ( a ) Mdr by E. coli expressing QacA or its D323C mutant. ( b ) pH dependence of multidrug resistance by E. coli UT mdfA::kan expressing MdfA or its V231E mutant. Resistance to Dmn and DAPI at pH 8 was tested at lower drug concentrations than pH 6.5 to make sure that even low-level resistance is not conferred. The experiments were repeated at least three times and the results shown are representative. Full size image Finally, as an independent complementary approach, we characterized the activity of MdfA(V231E). Unlike wild-type MdfA, this mutant is able to translocate two protons per transport cycle [8] , rendering it active against both LDCs and SDCs (as QacA) ( Fig. 9b , upper panel). If MdfA(V231E) exports LDCs in two successive cycles, in exchange for 2 protons per cycle (a total of 4 protons), the antiport would be electrogenic. In contrast, this mutant might catalyse electroneutral SDC/proton antiport, as these compounds are exported in a single cycle in exchange for two protons. To assess this prediction in vivo , we tested the pH dependence of MdfA(V231E) resistance activity against dications. The results show that this mutant could not confer resistance against SDCs (DAPI and Dmn) at elevated pH, suggesting electroneutral transport of these drugs (exchange of two protons per one dicationic substrate) ( Fig. 9b , lower panel). In contrast to SDCs, MdfA(V231E) conferred resistance against LDCs (Chx and Dq) even at pH 8 ( Fig. 9b , lower panel), suggesting that their transport is indeed electrogenic. When considered in the context of our hypothesis that LDCs are transported in two consecutive cycles, the indication that even in the absence of ΔpH the mutant can energize Dq efflux suggests that the transport is likely to be electrogenic and each of the two positive moieties of Dq might be exchanged for two protons. Together, the results suggest that MdfA(V231E) catalyses efflux of LDCs with an overall higher proton exchange stoichiometry than SDCs, in support of the hypothesis that LDCs are exported by MFS secondary Mdr transporters in two consecutive cycles. Recently, important aspects of the mechanism underlying MdfA-mediated antiport were elucidated [4] . A key principle in the mechanism is that substrate binding triggers release of a single stoichiometric proton from MdfA. This offers an explanation for the proton/drug antiport stoichiometry of 1 that was observed with MdfA [5] . Different MFS Mdr transporters work with distinct proton antiport stoichiometries. For example, QacA from S. aureus and LmrP from L. lactis use stoichiometries of up to 2 or 3 (refs 6 , 7 ). Compared with most Mdr transporters, the proton/drug stoichiometry of 1 (as shown for MdfA) is relatively low, rendering it generally inactive in efflux of dicationic drugs [8] . Indeed, MdfA mutants that are capable of pumping two protons per drug molecule acquire resistance also against dicationic drugs [8] . Therefore, in the case of wild-type MdfA, the discovery of efflux of certain dicationic drugs (LDCs) was surprising and posed a mechanistic riddle. An important clue to solving this was that MdfA seems to confer resistance only to LDCs, whose two positive charges are separated by a long linker. Our studies showed that LDCs are transported in a manner similar to the monocationic drugs. Namely, they are exchanged with protons, bind the transporter with a 1:1 stoichiometry and, most importantly, their transport is electroneutral. This suggests that they are probably exchanged for two protons. Nevertheless, binding of LDCs induces the release of only a single proton from MdfA, just like monocationic drugs [4] . If so, why is their proton/drug antiport stoichiometry twice higher? The unique architecture of these substrates, with two charges that are separated by a long linker, offers a hypothetical solution. We propose that MdfA exports LDCs in two successive transport cycles, in which each charged moiety is transported as if it were a separate substrate. In each cycle, one proton is transported, thus providing a total of two protons imported during the process, which ends after the full release of the LDC molecule from MdfA. According to this scenario, the carbon chain that separates the two charged domains of the LDCs must remain buried inside the transporter, or in the lipid-transporter interface, just before the second transport cycle ( Fig. 8 ). Such a hydrophobic linker may behave as a carbon chain of lipids and integrate into the lipid–protein structure without interrupting the ability of MdfA to undergo transport-related conformational changes. Through additional studies with QacA and its D323C mutant and with the MdfA mutant V231E, we obtained evidence in support of the proposed mechanism and the notion that it might be universal in secondary Mdr transporters. Briefly, the results show that QacA(D323C), which is in principal a monocationic drug pump, can confer resistance against LDCs. Furthermore, we showed that an MdfA mutant that generally exchanges two protons per dicationic drugs from the SDC group can transport also LDCs; however, these compounds are exchanged for more than two protons. This is consistent with the hypothesis that LDCs are transported in two sequential cycles also by this MdfA mutant. It seems that the simplest explanation for these observations is that MFS Mdr transporters handle certain dicationic drugs as if they were two separate monocations, which are transported separately. Transport of a substrate in more than a single cycle has never been demonstrated for secondary or primary active solute transporters. Transported substrates are usually small molecules that do not justify such a mechanism, because they can be transported in a single step. Transport of larger molecules, such as proteins across the membrane is usually catalysed by machineries that generate a continuous transmembrane channel [24] . The continuous channel enables such large substrates to be transported in a step-wise, processive manner. In active transporters, the substrate-conducting channel is always blocked on either side of the membrane. The transport mechanism works such that when the blockade is opened on one side, it closes on the other side of the membrane, enabling the substrate to bind or dissociate from either side of the membrane alternatively. This blockade should hinder processive transport; however, our results suggest that relatively narrow, hydrophobic linkers may still be threaded through the blocked channel. This mechanism might be shared by other active transporters that translocate large substrates with long linkers. The unusual processive mechanism broadens the substrate profile of Mdr transporters and may extend the spectrum of substrates that are accessible for active transporters in general. Drug resistance assay Antibacterial resistance was assayed as described [25] . Briefly, E. coli UT mdfA::Kan or UTL2 mdfA::Kan [25] harbouring empty vector or expressing MdfA were grown aerobically to A 600 of 1 and a series of 10-fold dilutions was prepared. Four microlitres of the serial dilution were spotted on drug-containing LB-agar plates and tested for growth after overnight incubation at 37 °C. pH-dependent resistance was tested by adding 75 mM bis-Tris-propane buffer at the indicated pH to the media as described [5] . Resistance conferred by QacA was assayed similarly with the following modifications: (i) the E. coli strain used was DH5α; (ii) the control vector was pBluescriptII, on which the plasmids encoding QacA (pSK4322) and QacA(D323C) (pSK4432) are based; (iii) liquid cultures were grown in 2YT media supplemented with 0.1 mg ml −1 ampicillin. All drugs were from Sigma Aldrich. MdfA overexpression and purification E. coli cells harbouring plasmid pUC18/ Para / mdfA - His6 were grown at 37 °C in LB medium supplemented with ampicillin (200 μg ml −1 ). Overnight cultures were diluted to 0.07 A 600 units, grown to 1.0 A 600 units and induced with 0.2% arabinose for 1 h. A typical 10-l culture yielded 15 g (wet weight) of cells. Cell pellets were washed once in 150 ml of 50 mM KPi (pH 7.3) supplemented with 5 mM MgSO 4 and collected by centrifugation (10 min, 10,000 g ). Next, the cells were suspended in 150 ml of the same buffer containing 10 μg ml −1 DNAse and 1 mM phenylmethylsulphonyl fluoride and passed three times through a liquidizer (Emulsiflex-C5, Avestin) (10,000 psi) for disruption. Cell debris was removed by centrifugation (30 min, 10,000 g ) and the membranes were collected by ultracentrifugation (1 h, 100,000 g ). The membranes were homogenized in 27 ml of urea buffer (20 mM Tris-HCl pH 8, 0.5 M NaCl, 5 M urea, 10% glycerol, 28 mM β-mercaptoethanol and 1 mM phenylmethylsulphonyl fluoride), incubated for 30 min at 4 °C and collected by ultracentrifugation (2.5 h, 100,000 g ). The membranes were washed with 27 ml of membrane buffer (20 mM Tris–HCl pH 8, 0.5 M NaCl, 10% glycerol and 3.5 mM β-mercaptoethanol). Finally, the membranes were suspended by homogenization in 7 ml of the same buffer and aliquots of 1 ml were snap-frozen in liquid nitrogen and stored at −80 °C. For MdfA purification, thawed membranes were diluted fivefold in solubilization buffer (20 mM Tris–HCl pH 8, 0.5 M NaCl, 10% glycerol, 0.1% β-dodecyl maltopyranoside (DDM), 5 mM imidazole) and solubilized by gradual addition of 10% DDM (Anatrace) to a final concentration of 1.1% and homogenized. Insoluble material was discarded by ultracentrifugation (30 min, 100,000 g ) and the soluble fraction was mixed with solubilization buffer-equilibrated Talon beads (Clontech) (typically 0.5 ml for 2 ml of thawed membranes). Next, the mixture was agitated for 3 h at 4 °C and the suspension was poured into a column. The column was then washed twice with ten-column volumes of solubilization buffer. MdfA was eluted in elution buffer (20 mM Tris–HCl pH 7.2, 0.12 M NaCl, 10% glycerol, 0.1% DDM, 100 mM imidazole). The protein was collected after initial discard of 0.75 column volume. The protein was then dialysed overnight against dialysis buffer (20 mM Tris-HCl pH 7.2, 0.12 M NaCl, 10% glycerol, 0.01% DDM) at 4 °C. Protein concentration was determined by measuring A 280 (1 mg ml −1 ~2.1 A 280 ) [13] . Measurement of [ 3 H]-TPP binding Radiolabelled TPP binding was carried out by immobilizing purified MdfA-His 6 on Ni 2+ beads, allowing it to bind [ 3 H]-TPP (American Radiolabeled Chemicals) and counting the MdfA-associated radioactivity as described [13] . For assessment of competition, the indicated concentrations of competitors were added during [ 3 H]-TPP binding. To determine K I , the data were fitted to the equation B = B max − B max × ([Dq]/([Dq+ K I )) using nonlinear regression, where B is the amount of bound [ 3 H]-TPP (in counts) and B max is the maximal amount of B (without added Dq). Dq transport in whole cells Overnight cultures of E. coli UTL2 mdfA :: kan cells harbouring empty vector (pT7-5) or plasmid pT7-5/ mdfA-His 6 were diluted 50-fold and grown at 37 °C in LB broth supplemented with ampicillin (100 μg ml −1 ) and kanamycin (30 μg ml −1 ) up to an A 600 of ~1 and transferred to ice. Ice-cold cell suspensions (0.3 A 600 units) were pelleted and washed once with 1 ml of wash buffer (50 mM KPi pH 7, 0.2% glucose, 2 mM MgSO 4 ), centrifuged and resuspended in 110 μl of the same buffer. From these cells, 100 μl were added to a cuvette containing 1,900 μl of pre-warmed (37 °C) wash buffer supplemented with 1 μM Dq (Sigma). The suspension was continuously stirred and warmed while measuring Dq fluorescence quenching (excitation 330 nm, emission 370 nm). For experiments with CAM, the wash buffers were supplemented with 0.8 mM CAM (Sigma). For dissipation of ΔpH, the protocol was modified as follows: cell suspensions were pelleted, resuspended and incubated for 10 min in modified wash buffer (50 mM KPi pH 8, 1% EtOH, 2 mM EDTA, 2 μM nigericin (Fermentek)). Cells were centrifuged and resuspended in 110 μl of the same buffer. From these cells, 100 μl were added to cuvette containing 1,900 μl of pre-warmed (37 °C) modified wash buffer supplemented with 1 μM Dq and 0.2% glucose, and the fluorescence was recorded. Estimation of Dq fluorescence inside cells was done similarly with modifications. Cells ( A 600 of 1.5) were pelleted and resuspended in 100 μl wash buffer. To this suspension, 1.5 ml of Dq-supplemented wash buffer was added and the cells were allowed to accumulate Dq for 0 or 14 min at 37 °C. Cells were centrifuged (1 min, 13,000 r.p.m., tabletop centrifuge, Eppendorf 5424) immediately after incubation and the supernatant was discarded. Pellets were resuspended in 100 μl water, mixed with 1.5 ml of 1% SDS and incubated at ambient temperature for several minutes. Dq fluorescence in these lysates was determined fluorimetrically. Proton transport in everted membrane vesicles Proton antiport was assayed as described [4] . E. coli UT5600/ mdfA::kan cells overexpressing MdfA (from plasmid pT7-5/ araP/mdfA-His6 ) or harbouring empty vector were grown to A 600 of ~1.2, induced for 1 h by arabinose and everted membrane vesicles were prepared as described [26] . Membranes were frozen by liquid N 2 in 10% glycerol, 5 mM MgSO 5 , 50 mM KPi pH 7.3 in a concentration of 20 mg ml −1 protein and stored at −80 °C. Membranes were thawed quickly at 46 °C for experiments. For each measurement, 20 μl membranes were diluted into 2 ml of pre-warmed (30 °C) proton transport solution (50 m mM K-gluconate, 50 mM KCl, 10 mM MgSO4, titrated to pH 6 and supplemented with 1 μM ACMA (Sigma-Aldrich)). Membranes were equilibrated for 4 min before fluorescence measurement (excitation and emission wavelengths of 409 and 474, respectively). The samples were continuously stirred during measurement. At the indicated times, D,L -lactate (2 mM), drugs (at the indicated concentrations) or carbonyl cyanide m -chlorophenyl hydrazone (0.01 μM, Sigma-Aldrich) were added. Lactate stocks (200 mM) were titrated with NaOH to pH 7 before experiments. Measurement of substrate-induced proton release Proton release was measured as described [4] . Purified MdfA was dialysed 4 times against 100 volumes of unbuffered solution containing 120 mM NaCl, 10% glycerol and 0.01% DDM. The protein was diluted to 2 μM in 120 mM NaCl, 10% glycerol, 0.1% DDM and 1 μM fluorescein was added. The mixture was titrated to fluorescence of ~550 (pH~6.5) before the experiment. During the experiment, the fluorescence was measured (excitation and emission wavelengths of 488 and 513, respectively), while samples were continuously stirred at ambient temperature. Substrates were added at concentrations of 150 μM (TPP), 50 μM (Dq) or 300 μM (Pent). HCl was added at a concentration of 2 μM. Dq binding measured by fluorescence Purified MdfA was concentrated using Vivaspin ultrafiltration spin columns (100 kDa cutoff, Sartorius). MdfA and Dq were mixed at concentrations of 10 μM MdfA and 0.2 μM Dq. Next, this mixture was serially diluted (1.42-fold each dilution) into a solution containing only 0.2 μM Dq, keeping [Dq] constant while diluting MdfA. The fluorescence of each increasingly diluted sample was measured in a quartz cuvette (excitation and emission wavelengths of 330 and 370, respectively). To determine K d , the data were fitted to the equation: fluorescence (%)=100%−((Δ F × [MdfA])/( K d +[MdfA])) using nonlinear regression, where Δ F is the percent fluorescence difference upon MdfA binding. Dq-mediated cross-linking of MdfA Everted membrane vesicles were prepared from cells overexpressing MdfA or the functional split mutant N8-His 6 /C4-His 6 (ref. 20 ) as described above for proton transport measurements. Membrane vesicles were thawed, collected by ultracentrifugation (100,000 g , 30 min, 4 °C) and resuspended in 0.5 M NaCl, 10% glycerol, 20 mM Tris-HCl pH 8 at a total protein concentration of 1 mg ml −1 . Dq (100 μM final) or buffer was added to 40 μl vesicles and was allowed to bind during 20 min incubation at ambient temperature in the dark. Samples were transferred to ice-cold 96-well plates and irradiated on ice for 20 min with ultraviolet at 366 nm from a distance of 2.7 cm using Model UVGL-25 Minervalight lamp (San Gabriel, CA). Irradiated samples (40 μl) were mixed with 13.3 μl 4 × protein sample buffer and 10 μl samples were analysed by SDS–PAGE and western blotting as described [4] . How to cite this article: Fluman, N. et al . Export of a single drug molecule in two transport cycles by a multidrug efflux pump. Nat. Commun. 5:4615 doi: 10.1038/ncomms5615 (2014).